Large magnetocaloric effect and adiabatic demagnetization refrigeration with YbPt2Sn Adiabatic demagnetization is currently gaining strong interest in searching for alternatives to 3 He-based refrigeration techniques for achieving temperatures below 2 K. The main reasons for that are the recent shortage and high price of the rare helium isotope 3 He. Here we report the discovery of a large magnetocaloric effect in the intermetallic compound YbPt 2 Sn, which allows adiabatic demagnetization cooling from 2 K down to 0.2 K. We demonstrate this with a home-made refrigerator. Other materials, for example, paramagnetic salts, are commonly used for the same purpose but none of them is metallic, a severe limitation for low-temperature applications. YbPt 2 Sn is a good metal with an extremely rare weak magnetic coupling between the Yb atoms, which prevents them from ordering above 0.25 K, leaving enough entropy free for use in adiabatic demagnetization cooling. The large volumetric entropy capacity of YbPt 2 Sn guarantees also a good cooling power. Usage of 3 He is found in a variety of fields encompassing medical applications, military purpose and scientific research [1] , [2] , [3] . In science and engineering, 3 He is one of the essential ingredients to achieve very low temperatures [4] or to detect radioactivity [1] . We experience today a period of supply cutbacks for miscellaneous demands and very high costs for pure 3 He: For example, low-temperature physicists have required only 1.3% of the available 3 He between 2004 and 2010, and the price rose by a factor of 15 (refs 2 , 3 ). Before this cutback, they were the major consumers of 3 He, since temperatures down to 0.3 K and below were mostly reached by 3 He systems and 3 He/ 4 He dilution refrigerators [4] . Given that 3 He has been solely obtained as a byproduct from decay of tritium in nuclear weapons stockpiles or nuclear reactors, global agreement to reduce those facilities still holds, it seems unlikely to generate a smooth supply of 3 He in the future. Consequently, we are now obliged to search alternatives to circumvent this 3 He crisis. Fortunately, low-temperature physicists already developed a 3 He-free system, the adiabatic demagnetization refrigerator (ADR). This device makes use of magnetocaloric materials (MCMs) which are essentially paramagnetic compounds [5] . The term magnetocaloric was reported for the first time by Weiss and Piccard [6] , and the magnetocaloric effect (MCE) has been defined as reversible adiabatic variation in temperature of a material by an applied magnetic field. Compared with cumbersome gas-handling for 3 He containing fridges, ADRs provide much easier operation: simple ramping-up and -down a magnet while operating (opening) a heat-switch cools down the system (see later). But further development of ADRs was delayed due to widespread adoption of the dilution refrigerator since the 1970s, because of its specific continuous cooling capacity. Although continuous cooling is also available in ADR since the initiation of space projects requiring zero-gravity cryostats [7] , [8] , most popular MCMs at low temperatures are still the paramagnetic salts which were independently proposed by Debye and Giauque [9] , [10] , [11] 80 years ago. Until recently, the MCE was best known for the working principle of ADR but it has also yielded invaluable information about magnetic phase transitions [12] , quantum criticality [13] , [14] , [15] and alternative refrigeration techniques [16] , [17] in modern science. An ideal MCM for low-temperature applications should be made of magnetic atoms, which are in a degenerate paramagnetic state down to the lowest possible temperature in zero magnetic field. Then, it should have a large volumetric entropy capacity for a good cooling power. In addition, it is preferred to be metallic and non-superconducting for better conduction of heat and easy machining. And finally, it should not degrade over time. So far, most of the materials used for temperatures below 2 K have only fulfilled the first two requirements [7] , but sophisticated treatments are mandatory to meet the standard of operation: To protect the MCMs and for a sufficient thermal contact, those non-metallic MCMs must be prepared inside a canister with special metallic structures [18] , [19] . In this article, we demonstrate that the metallic compound YbPt 2 Sn, which satisfies all aforementioned prerequisites for a MCM at low temperatures. We have measured the specific heat capacity C ( T , B ) of polycrystalline YbPt 2 Sn [20] down to a temperature T =0.05 K and magnetic field B up to 7 T by using a compensated heat-pulse method [21] . The entropy S ( T , B ) converted from C ( T , B ) is used to estimate the MCE and the minimum temperature accessible by adiabatic demagnetization, which results to be <0.2 K. Finally, we show a direct measurement of the MCE performed in a home-made ADR with an YbPt 2 Sn ingot and demonstrate how an ADR made with YbPt 2 Sn is a feasible and durable alternative to 3 He-cryostats. Specific heat of YbPt 2 Sn The relevant actors in our study are the Yb 3+ ions, which are in the magnetic 3+ valence state with total angular momentum J =7/2. They are exposed to a crystalline electric field (CEF) with hexagonal symmetry, which lifts the degenerate 4 f -shell energy levels into four doublets leaving a Kramers doublet as ground state with effective spin 1/2 and maximum entropy R ln2=5.76 J K −1 mol −1 (with R the gas constant) [20] . This is best shown in Fig. 1a , where the specific heat capacity C ( T , B ) of YbPt 2 Sn is plotted over a broad range of temperatures 0.06 T 200 K and at selected magnetic fields 0 B 7 T. We start to look at C / T in zero field (black symbols). At high temperatures, C / T displays two broad maxima, at about 50 and 6 K, which are due to phonons and a Schottky peak caused by thermal occupation of the first excited CEF level, respectively. Below 3 K, C / T increases steeply with a 1/ T 2 dependence which is attributed to the emergence of short-range (intersite) magnetic correlations, which are not sufficient to induce long-range magnetic ordering [20] . Eventually, at T m =0.25 K short-range magnetic ordering sets in and is manifested as a kink in C ( T )/ T , similar to the parent compound YbPd 2 Sn [22] . Such a low T m is very uncommon in Yb-based intermetallic systems with no sizeable Kondo interaction (like YbPt 2 Sn), which usually have transition temperatures of a few Kelvin. The nature of the magnetic ordering and the reason for the very weak magnetic exchange (≈0.8 K (ref. 20 )) are still unknown, but this unique behaviour allows us to use the full unquenched entropy between T m and 4 K for AD cooling in the same T -range of 3 He systems. 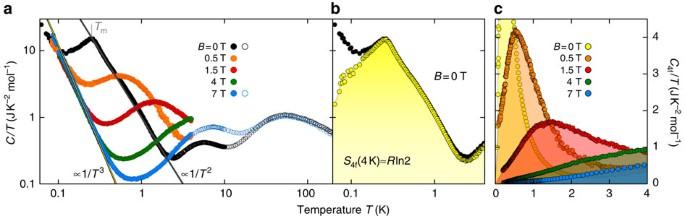Figure 1: Specific heat of YbPt2Sn. (a)T-dependence of the specific heat capacity of YbPt2Sn divided by the temperature,C/T, at different magnetic fields in a double-logarithmic plot. Empty and filled symbols are data obtained with a standard4He-cryostat and a dilution refrigerator, respectively. The straight lines emphasize the 1/T2increase ofC/Tdue to strong fluctuations and the typical 1/T3dependence ofC/Tfor the high-temperature side of the nuclear Schottky peak.Tm=0.25 K marks the onset of the short-range magnetic ordering. (b) 4f-electron contributionC4f/T(yellow symbols) to the total specific heatC/T(black symbols) atB=0 after having subtracted the conduction-electron contributionγ=0.03 J K−2mol−1and the nuclearαn/T3contribution withαn=5.8 mJ K mol−1(seeSupplementary Fig. 1andSupplementary Note 1). The yellow area under theC4f/TversusTcurve is the entropy released up to 4 K, S4f(4K)≈Rln2, the maximum entropy for a doublet ground state. (c)C4f/TversusTatB=0, 0.5, 1.5, 4 and 7 T. Figure 1: Specific heat of YbPt 2 Sn. ( a ) T -dependence of the specific heat capacity of YbPt 2 Sn divided by the temperature, C / T , at different magnetic fields in a double-logarithmic plot. Empty and filled symbols are data obtained with a standard 4 He-cryostat and a dilution refrigerator, respectively. The straight lines emphasize the 1/ T 2 increase of C / T due to strong fluctuations and the typical 1/ T 3 dependence of C / T for the high-temperature side of the nuclear Schottky peak. T m =0.25 K marks the onset of the short-range magnetic ordering. ( b ) 4 f -electron contribution C 4 f / T (yellow symbols) to the total specific heat C / T (black symbols) at B =0 after having subtracted the conduction-electron contribution γ =0.03 J K −2 mol −1 and the nuclear α n / T 3 contribution with α n =5.8 mJ K mol −1 (see Supplementary Fig. 1 and Supplementary Note 1 ). The yellow area under the C 4 f / T versus T curve is the entropy released up to 4 K, S 4 f (4 K )≈ R ln2, the maximum entropy for a doublet ground state. ( c ) C 4 f / T versus T at B =0, 0.5, 1.5, 4 and 7 T. Full size image At T < T m , C / T increases again as 1/ T 3 because of the nuclear contribution C n to the specific heat from the nuclear moment of Yb, see Supplementary Fig. 1 and Supplementary Note 1 . This is emphasized by the measurements at different fields where the 1/ T 3 increase does not change much with B but becomes more visible. In fact, increasing B rapidly suppresses the phase transition at T m . The kink at T m transforms into a Schottky peak, which shifts to higher T , uncovering the large increase of C n / T below 1 K. This Schottky peak is the result of the Zeeman splitting of the ground state doublet and is the fundamental effect needed for the MCE. To demonstrate this we have subtracted from all C ( T )/ T curves the small conduction-electron contribution C e / T ( T →0)= γ and the nuclear contribution C n / T = α n / T 3 to obtain the pure 4 f -electron specific heat C 4 f (see Supplementary Fig. 1 and Supplementary Note 1 ). In this temperature range, the phonon contribution is negligible. For B =0 the results are shown in Fig. 1b with γ =0.03 J K −2 mol −1 and α n =5.8 mJ K mol −1 (yellow symbols). Now, evaluating the 4 f -electron entropy S 4 f from the integral of C 4 f / T between 0.06 and 4 K ( cf. yellow area in Fig. 1b ), we obtain exactly R ln2, the maximum entropy for a doublet ground state. Increasing the field results in a shift of this entropy to higher T , as shown in Fig. 1c (coloured areas), inducing the MCE we are after. Entropy and MCE By integrating C 4 f / T for all fields we can extract the full 4 f -electron entropy S 4 f ( T , B ). To investigate useful adiabatic paths, we have generated a surface plot interpolating the S 4 f ( T , B ) curves, which is shown in Fig. 2a . As a result, the coloured surface clearly exhibits a notable MCE: The isothermal suppression of entropy (black arrow) followed by the isentropic trace (red arrow) allows to decrease the temperature. T i and T f designate the initial and the final temperature. The same is illustrated in Fig. 2b , that is, the projection of the data into the S – T plane. In Fig. 2c , we have plotted the expected T f of YbPt 2 Sn as a function of T i marked in Fig. 2a . The lower T i the lower T f . T f is further decreased as we suppress the entropy with stronger field. It is clear that this material can always be cooled down below 0.2 K, in a reasonable range of T and B for a standard 4 He-cryostat and a superconducting magnet. This is because the transition at T m does not quench much of the entropy and the MCE allows to cool down the system below T m . However, while theory suggests that it should be possible to cool down well-below 0.2 K, in real experiments (see below and Supplementary Fig. 3 ), only temperatures slightly below 0.2 K were achieved. 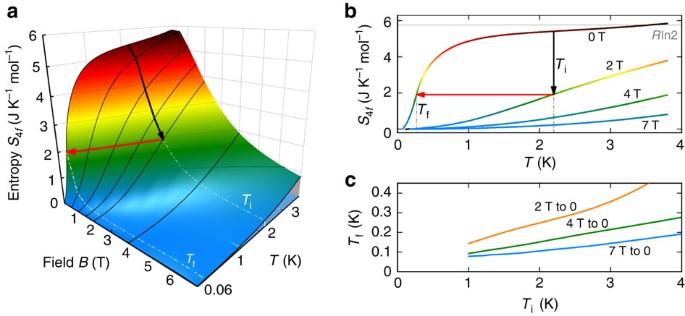Figure 2: Magnetic entropy and magnetocaloric effect of YbPt2Sn. (a) Colour map of the 4f-electron magnetic entropy,S4f(T,B)=(C4f/T)dT, of YbPt2Sn. Black solid lines are calculated from the measuredC4f(T,B)/Tand the coloured surface is an interpolation of the data. Regions with the same colour are isentropic. The black arrow designates the isothermal suppression of the entropy, and the red arrow designates the adiabatic demagnetization revealing a clear MCE. (b) Projection into theS–Tplane of the data. The grey line marksRln2, which is the saturation entropy of the ground state doublet. (c) Initial temperatureTidependence of the final temperatureTffor different adiabatic traces or isentropic contours. Figure 2: Magnetic entropy and magnetocaloric effect of YbPt 2 Sn. ( a ) Colour map of the 4 f -electron magnetic entropy, S 4 f ( T , B )=( C 4 f / T ) dT , of YbPt 2 Sn. Black solid lines are calculated from the measured C 4 f ( T , B )/ T and the coloured surface is an interpolation of the data. Regions with the same colour are isentropic. The black arrow designates the isothermal suppression of the entropy, and the red arrow designates the adiabatic demagnetization revealing a clear MCE. ( b ) Projection into the S – T plane of the data. The grey line marks R ln2, which is the saturation entropy of the ground state doublet. ( c ) Initial temperature T i dependence of the final temperature T f for different adiabatic traces or isentropic contours. Full size image There are several materials, like paramagnetic salts or magnetic garnets (see Table 1 ), which are used for AD cooling in the same temperature range, but the advantage of YbPt 2 Sn is that it is a good metal and it can easily be cast into rods, making preparation of cooling pills quite simple, in contrast to salts or garnets. To test our material, we built a simple home-made ADR with a 10 g ingot pillar of YbPt 2 Sn (shown in Fig. 3c ). More details will be found in Methods: ADR set-ups. Direct measurements of the MCE with the YbPt 2 Sn ingot are shown in Fig. 3a . Along the path from 6 T (red line), starting at 1.45 K, with a sweep rate of 0.1 T min −1 , the temperature of the pillar, T pillar , had reached 0.19 K, which is about 0.1 K higher than the T f estimated from Fig. 2 . After that, the pillar began to warm up due to inevitable heat loads from the electrical wiring and supporting structures ( cf. Fig. 3b ). The magnet power supply was the source of oscillations and occasional spikes in T pillar ( B ). Another adiabatic path from 4 T, starting from 1.75 K with higher sweep rate of 0.13 T min −1 ended at 0.22 K, which is also 0.1 K higher than the estimated T f . The uppermost cycle shows a ramping-up from 0 T and 0.26 K to 2 T and 1.3 K, and a successive ramping-down to 0 T and 0.27 K after 1 h of intermission. Also here, the 0.27 K achieved by MCE from 2 T and 1.3 K is about 0.1 K higher than the estimation. The discrepancy between T pillar (0) and T f is reasonable given that thermal and mechanical insulations were not as good as in a commercial standard ADR. In fact, the Kapton tubes guarantee good thermal insulation only below 1 K. We have also tested YbPt 2 Sn in a commercial physical properties measurement system (PPMS) (Quantum Design) by using an even simpler design without a heat-switch (see Supplementary Figs 2 and 3 ) and reached about 0.16 K. However, our experimental set-up provided a good enough thermal insulation at the lowest temperatures, which is reflected in a warming-up rate of 0.01 K h −1 at about 0.2 K, as shown in Fig. 3b . The reversibility and linearity of T pillar ( B ), regardless of the sweep rate, indicates negligible eddy-current heating (see green curves in Fig. 3a ). Consequently, the MCE observed in YbPt 2 Sn is reminiscent of that of an ideal paramagnet. An ideal paramagnet is universally described by ( T / B ) S =( T / B ) and T f = T i ( B f / B i ) regardless of material parameters, where B i and B f are the initial and final magnetic fields along an adiabatic path, respectively. This means that at B f =0, T f =0. This is not the case for YbPt 2 Sn where we observe a finite T f = T pillar (0)≈0.2 K at B f =0 (see black straight lines in Fig. 3a ). This is certainly due to the magnetic weak exchange interaction, which is of the same order of magnitute of T pillar (0) and T m (ref. 20 ). Table 1 Comparison of parameters for various magnetocaloric materials. 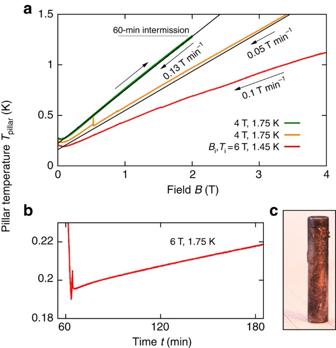Figure 3: Realization of AD cooling with YbPt2Sn. (a) Measurements of the MCE by means of quasi-adiabatic demagnetization. The temperature of the YbPt2Sn ingot pillar (photograph),Tpillar, is shown for various paths. Current record of the lowest temperature is 0.19 K, which was reached starting from 6 T and 1.45 K. From 4 T and 1.75 K, 0.22 K was reached and few hours later the temperature rose to 0.26 K. From this point, the pillar was magnetized up to 2 T and held for 1 h before it was demagnetized again. Arrows alongside each measurements indicate the directions of the sweeps and the sweep rates are also noted nearby. Almost a linear behaviour of the measuredTpillar(B) emphasized by the straight lines is evidence of the paramagnetic MCE. (b) Increasing ofTpillarwith time: about 0.01 K h−1. (c) The ingot pillar (10 g) of YbPt2Sn. Full size table Figure 3: Realization of AD cooling with YbPt 2 Sn. ( a ) Measurements of the MCE by means of quasi-adiabatic demagnetization. The temperature of the YbPt 2 Sn ingot pillar (photograph), T pillar , is shown for various paths. Current record of the lowest temperature is 0.19 K, which was reached starting from 6 T and 1.45 K. From 4 T and 1.75 K, 0.22 K was reached and few hours later the temperature rose to 0.26 K. From this point, the pillar was magnetized up to 2 T and held for 1 h before it was demagnetized again. Arrows alongside each measurements indicate the directions of the sweeps and the sweep rates are also noted nearby. Almost a linear behaviour of the measured T pillar ( B ) emphasized by the straight lines is evidence of the paramagnetic MCE. ( b ) Increasing of T pillar with time: about 0.01 K h −1 . ( c ) The ingot pillar (10 g) of YbPt 2 Sn. Full size image How good is YbPt 2 Sn compared with standard MCM materials for the same T -range? In a MCM, a weak magnetic interaction is beneficial to achieve a low base temperature. Moreover, the spin J GS of the ground state determines the saturation entropy R ln(2 J GS +1) and, therefore, a large J GS is advantageous for a stronger cooling power. It is worth mentioning that for practical purposes it is not the molar entropy but it is the entropy density of the material which is the relevant quantity. Finally, a large g -factor is desirable because the suppression of entropy by a magnetic field becomes more susceptible. Hence, for a MCM large J GS , g , density d and a weak magnetic interaction are desirable, but large values of the first three parameters promote a strong magnetic interaction. Thus creating a low-temperature magnet with a weak interaction usually is in conflict with having a large cooling capacity and vice versa . Table 1 shows relevant parameters for paramagnetic salts and garnets, which are popular MCMs for ADR <1 K. In chromium potassium alum and ferric ammonium alum, first order magnetic phase transitions appear near T m ≈10 mK (ref. 23 ) and T m ≈30 mK (ref. 24 ), respectively. Normally, the ordering temperature T m is indicative of the lowest possible temperature as entropy is quenched with a phase transition. As mentioned above, the intuitive approach to keep large distance between magnetic ions to obtain low T m (typical of these materials) is accompanied by the downside of having low volumetric entropy capacity, S v . For gadolinium gallium garnet [25] and dysprosium gallium garnet [26] , one can have much higher S v than salts at the expense of T m . Moreover, it is common to have higher T m as J GS is increased [27] . In comparison to salts, YbPt 2 Sn has more than eight times larger d , and roughly three times larger S v while it orders at 0.25 K. At first glance, the tendency to relinquish a low T m over S v seems to be obeyed. However, in contrast to rare-earth garnets and other rare-earth MCMs [28] , the magnetic ordering around 0.2 K cannot be accounted for by neither J GS nor d dependence. Most of all, the weak and continuous magnetic ordering makes YbPt 2 Sn unique because it can be practically cooled below T m . It is also worth noting that similar compounds like YbPd 2 Sn (with T m =0.23 K (refs 22 , 29 )) and YbPt 2 In (with T m =0.18 K (ref. 20 )) all show doublet ground states and weak ordering, but YbPd 2 Sn becomes superconducting at 2.3 K (that is, a bad thermal conductor) and YbPt 2 In has not yet been tested. It is worth mentioning that there are materials which show maximal MCE at the verge of metamagnetic transitions [30] . However, those materials require a demagnetization towards a nonzero field and the small entropy change would provide a weaker cooling effect when compared with that of YbPt 2 Sn. The aforementioned exceptional properties of YbPt 2 Sn allowed us to build an ADR with a metallic MCM operable below the base temperature of a 3 He-cryostat. This material can be easily cast into various shapes and directly attached to the cooling target without any complications. It is a good metal and no additional metallic structures are needed for the thermal conduction unlike in paramagnetic salts or garnets, which are very poor thermal conductors <1 K. In this sense, while the physical origin of the weak interaction still needs to be clarified, it is an important feature that makes YbPt 2 Sn a viable new metallic refrigerant material for ADR. YbPt 2 Sn makes ADR more accessible by resolving complications of preparing non-metallic materials, which have been used since the 1930s. At the same time, it provides low enough base temperatures so that it can be chosen as an alternative to 3 He-cryostats. We hope that our discovery will accelerate low-temperature physicists to escape from the ongoing 3 He crisis. Material preparation Despite the high vapour pressure of divalent Yb metal, YbPt 2 Sn can easily be prepared in a standard arc-melting furnace by first reacting Yb with the low melting Sn and then adding Pt. Details are given in ref. 20 . The pillar used for the PPMS set-up (see Supplementary Fig. 2 ) and the rod for the home-made ADR were obtained by casting pre-reacted YbPt 2 Sn in an appropriate mould in an arc-melting furnace and in a commercial high-frequency casting system (see Supplementary Movie 1 ), respectively. Heat capacity Measurements of heat capacity have been carried out in a dilution refrigerator (Oxford Instruments) for temperatures 0.05 T 4 K and magnetic field B up to 7 T by using a compensated heat-pulse method described in ref. 21 . For T >2 K, the measurements were performed in a 7 T PPMS. ADR set-ups To test the cooling capability and MCE of YbPt 2 Sn, we have built two different refrigeration systems. One follows the standard structure of commercial ADR, which is equipped with a mechanical heat-switch, and the other is a simple miniaturized version without heat-switch that can be used in a commercial PPMS, as shown in Supplementary Fig. 2 . In the former set-up, we have modified a top-loading 1 K pot cryostat. The sample stage (thin brass disc) is fixed below the 1 K pot by using a pair of Kapton straws and is located at the stray-field compensation zone of the superconducting magnet. Beneath this stage, two thin brass rods are stretched to the magnet centre from opposite edges of the sample stage, and the end of each rod is joined perpendicular to each arms of ‘Φ’-shaped brass part. The mass of the whole brass structure is about 30 g. The YbPt 2 Sn ingot pillar shown in Fig. 3c is clamped at the centre of this thin metal piece. A push-pull manual actuator is used to activate the mechanical heat-switch. Further details and specifications of this set-up will be reported elsewhere. How to cite this article: Jang, D. et al . Large magnetocaloric effect and adiabatic demagnetization refrigeration with YbPt 2 Sn. Nat. Commun. 6:8680 doi: 10.1038/ncomms9680 (2015).